Giant ultrafast photo-induced shear strain in ferroelectric BiFeO3 Generation of strain using light is a key issue for future development of ultrasonic devices. Up to now, photo-induced GHz–THz acoustic phonons have been mainly explored in metals and semiconductors, and in artificial nanostructures to enhance their phononic emission. However, despite their inherent strong polarization (providing natural asymmetry) and superior piezoelectric properties, ferroelectric oxides have been only poorly regarded. Here, by using ultrafast optical pump–probe measurements, we show that photogeneration/photodetection of coherent phonons in BiFeO 3 ferroelectric leads, at room temperature, to the largest intensity ratio ever reported of GHz transverse acoustic wave versus the longitudinal one. It is found that the major mechanism involved corresponds to screening of the internal electric fields by light-induced charges, which in turn induces stress by inverse piezoelectric effect. This giant opto-acoustic response opens new perspectives for the use of ferroelectric oxides in ultrahigh frequency acoustic devices and the development of new GHz–THz acoustic sources. Recently, ultrafast light-generation of coherent acoustic waves in the giga–terahertz (GHz–THz) frequencies range is attracting much more attention for sensing nanostructures [1] , [2] , [3] , [4] , [5] , [6] , complex liquids or biological systems [7] , [8] , as well as for the fast manipulation of optical [9] , electronic [10] , [11] or magnetic properties [12] , [13] , [14] , [15] . Among the numerous studies investigating acoustic wave generation, most of them have been conducted in metals, semiconductors and nanostructures made of them. Several mechanisms and phenomena have been revealed, including thermoelastic coupling driven by hot carriers [16] , [17] , electrostriction [18] , [19] , electronic deformation potential (also called electronic pressure) [1] , [20] , [21] , as well as piezoelectric coupling [22] , [23] , [24] , [25] . Moreover, in most of these studies the photogenerated longitudinal acoustic (LA) phonon has a stronger amplitude than the shear or transverse acoustic (TA) one limiting the spectrum of applications of coherent acoustic waves. To overcome such drawback and enhance the amplitude of shear strain in regards to the longitudinal one, a broken symmetry—or anisotropy—is required [22] , [23] , [26] . 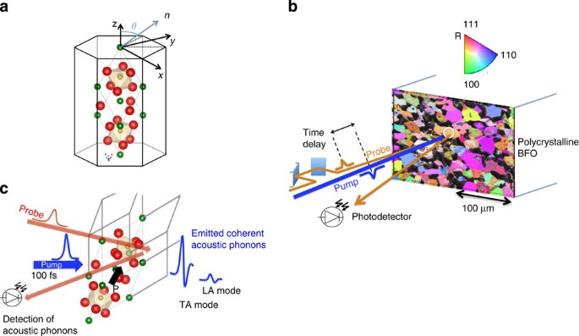Figure 1: Ultrafast pump-probe photoacoustic experiments on selected grains of polycrystalline ferroelectric BFO. (a) Unit cell of the rhombohedral structure of BFO where the red, green and yellow spheres correspond to oxygen, bismuth and iron atoms. The coordinates (x,y,z) are those employed for tensorial calculations, andzdirection corresponds to the polarization direction. (b) Schematic representation of the pump-probe experiment conducted onto a single grain of the polycrystalline sample with the white circle depicting the typical surface of the focused laser beam. The incident pump and probe beams are normal to the illuminated surface but slightly shifted off-normal in the figure, for clarity. The grain crystallographic orientations are revealed by the electron back scattering diffraction (EBSD) image obtained from Kikuchi patterns (each colour corresponds to a defined crystalline orientation in the rhombohedral (R) system, see Methods). (c) Principle of the ultrafast optical pump-probe experiments. The femtosecond pump light creates electron-hole pairs in the narrow band gap BFO that initiate the screening of the internal polarizationP, which in turn leads to the emission of coherent longitudinal (LA) and transverse (TA) acoustic phonons through the inverse piezo-electric effect. However, despite the many strategies to introduce such asymmetry in metals and semiconductors, the shear mode acousto-optic amplitude is at best of the same order of magnitude as that of the longitudinal phonon (see Table 1 ). Table 1 Comparison of different ultrafast TA mode photo-transducers. Full size table The search for alternatives to metals and semiconductors is therefore highly desired. Among possible candidates, ferroelectric oxides are of particular interest. Ferroelectrics possess a spontaneous polarization (switchable under application of an external electric field) issued from the loss of the inversion symmetry and thus asymmetry is naturally present. Interestingly, the typical polarization value is in the range of ~10–100 μC cm −2 and thus provides a strong inherent built-in potential able to efficiently separate photo-induced electron-hole carriers. Moreover, ferroelectrics are the strongest piezoelectric materials and as piezoelectric coupling provides a strong driving force for initiating coherent phonons, an efficient acoustic wave generation is expected. Among ferroelectric oxides, BiFeO 3 (BFO) has recently received a great deal of attention for its photo-induced effects [27] related to its small direct band gap ( E g =2.6–2.8 eV [28] ) enabling an efficient above band gap light absorption. As a result, in addition to its so-called multiferroic properties [29] (that is, simultaneous presence of polarization and magnetization), BFO has demonstrated various exotic properties, while not fully understood yet, when subjected to light including visible-light photovoltaic effect [30] , laser-induced ultrafast THz radiation [31] , [32] , giant electrochromic behaviour [33] , as well as photostriction properties [34] , with photo-induced lattice parameter expansion [35] , strain-modulated mosaicity [36] and ultrafast photogeneration of coherent acoustic phonons [37] , [38] . These recent findings demonstrate the potentiality of BFO as strain photogenerator. However, no studies related to the efficiency of the photogenerated TA and LA waves exist up to now. Moreover, although the direct link between the transient lattice strain and the electronic dynamics has been established [35] , the origin of the microscopic mechanisms driving the photo-induced strain, that is, piezoelectric [35] , [37] , [38] , [39] , electronic pressure [35] , [37] , [38] and electrostriction [34] , [38] effects, is still currently under debate and requires further investigations. Here we show that GHz coherent shear phonons can be photogenerated/photodetected in the ferroelectric oxide BFO with an efficiency that is estimated to be much higher than in any metals, semiconductors or nanostructures made of them. Interestingly, we found that using various crystallographic orientations of BFO lattice, the ratio between TA and LA amplitudes can be easily tuned, allowing to achieve a shear coherent acoustic mode with an acousto–optic amplitude more than five times larger than that of the longitudinal mode. Based on a detailed analysis of the data, we also discuss the mechanisms at the heart of the acoustic phonon generation in BFO. Mapping the grains orientation A bulk polycrystalline ceramic BFO sample with rhombohedral structure (R3c) shown in Fig. 1a is studied. The grains orientation is determined by electron backscattering diffraction (EBSD; see Methods). In the pump-probe technique used here we can then select by using appropriate light focalization conditions (beam size of tens of microns) a specific grain, that is, a single crystal of BFO with a given orientation, as shown in Fig. 1b , to study the ultrafast photogeneration process of coherent acoustic phonons as depicted in Fig. 1c . Note that as seen in Fig. 1b and in Supplementary Fig. 1 , the ceramic is poorly dense as the grains are separated by big holes (in black colour) allowing to assume that each grain is independent. Figure 1: Ultrafast pump-probe photoacoustic experiments on selected grains of polycrystalline ferroelectric BFO. ( a ) Unit cell of the rhombohedral structure of BFO where the red, green and yellow spheres correspond to oxygen, bismuth and iron atoms. The coordinates ( x , y , z ) are those employed for tensorial calculations, and z direction corresponds to the polarization direction. ( b ) Schematic representation of the pump-probe experiment conducted onto a single grain of the polycrystalline sample with the white circle depicting the typical surface of the focused laser beam. The incident pump and probe beams are normal to the illuminated surface but slightly shifted off-normal in the figure, for clarity. The grain crystallographic orientations are revealed by the electron back scattering diffraction (EBSD) image obtained from Kikuchi patterns (each colour corresponds to a defined crystalline orientation in the rhombohedral (R) system, see Methods). ( c ) Principle of the ultrafast optical pump-probe experiments. The femtosecond pump light creates electron-hole pairs in the narrow band gap BFO that initiate the screening of the internal polarization P , which in turn leads to the emission of coherent longitudinal (LA) and transverse (TA) acoustic phonons through the inverse piezo-electric effect. Full size image Ultrafast optical pump-probe study The pump-probe technique consists in the optical excitation of the system by a femtosecond laser pump beam and the detection of the corresponding transient optical reflectivity using a femtosecond laser probe beam (see Methods). More than 20 different grains have been studied and only some typical signals are shown in Fig. 2 . The transient optical reflectivity has been recorded up to a time delay of 2,000 ps and only a reduced time window is shown in Fig. 2a,c where long-living oscillations are clearly detected. The first strong peak at a time delay of 0 ps, also called electronic peak is related to the ultrafast electronic dynamics and has been already studied [40] . An appropriate fast Fourier transform reveals that depending on the grain considered, the oscillatory part contains up to three modes, that is, the quasi-longitudinal LA and the two quasi-transverse or shear TA1 and TA2 modes [37] . Note that as expected the frequency position depends on the orientation of the grain. The most striking and salient feature revealed in Fig. 2b,d is the appearance, for some grains, of spectacularly large coherent shear acoustic phonons signals (TA). However, for some grains ( Fig. 2f ), the TA modes are nearly absent. For the latter grains, the z axis of the unit cell (so-called optical axis) is nearly in plane of the irradiated surface. In that case, it is well known that a large optical birefringence is observed as previously reported [41] . In this particular situation, as we detect the acoustic phonons with circularly polarized light, the Brillouin LA mode is split into two modes, namely one detected by ordinary light and another by extraordinary light ( f o =37.3 GHz and f e =34.5 GHz). The ratio f e / f o of the Brillouin frequencies is in agreement with the ratio between the extraordinary and ordinary refractive indexes with f e / f o = n e / n o ≈0.92 (see Methods). On the contrary, for the other grains ( Fig. 2a–d ) with optical axes that are inclined, the birefringence is diminished as expected and appears only a little, for example, for the LA mode of grain 4. In a uniaxial medium (with z as the optical axis), there is indeed a direct relation linking the angle between the z axis and the surface normal that allows us to assess directly the grain orientation [41] . Furthermore, interestingly, the largest shear mode amplitude is obtained for a configuration where only one TA mode is observed (case of grains 2 and 3 in Fig. 2b,d ). All these ultrafast opto-acoustic signals indicate that for a given pump wavelength, the amplitude of the electronic excitation (called EE in Fig. 2a ), which can be estimated through the amplitude of the first peak of the transient reflectivity at t ~0 ps, is equivalent from grain to grain, but the acoustic signal (Brillouin oscillations marked as BO in Fig. 2a ) is drastically different. This observation indicates that a given population of photo-excited carriers couple differently to the lattice to emit coherent acoustic phonons. 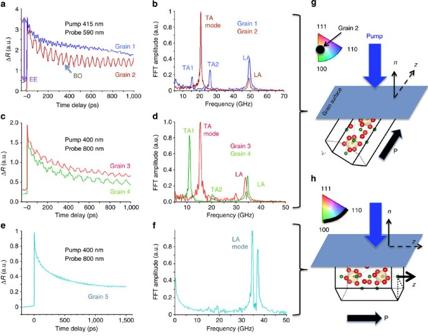Figure 2: Spectra of photogenerated longitudinal and TA modes for different crystallographic orientations. Transient optical reflectivity signals obtained for different grains of the polycrystalline BFO sample with pump (probe) wavelength of (a) 415 nm (590 nm) and (c,e) 400 nm (800 nm). The Brillouin oscillations (BO) are clearly visible. The Brillouin signal exhibits deep dependence on the grain while the electronic excitation (EE) is independent. (b,d,f) Plots of the corresponding fast fourier transforms of signals shown in (a,c,e). The grain 1–4 are inclined grains versuszaxis of the unit cell of BFO and show clear shear TA modes. (g,h) Sketches of the mean macroscopic polarizationPdirection relative to the grain surface normaln. The surface orientation of grain 2 is indicated on the mosaic (inset ofg) as an example. Grain 5 has itszaxis (called optical axis) parallel to the grain surface and TA modes are nearly absent, while LA modes are visible with a splitting due to optical anisotropy of BFO (see Methods). The family of planes, to which belongs the surface of grain 5, is indicated with the black line on the mosaic (inset ofh) (remark: the small signal at ~30 GHz for grain 3 is an artefact probably arising from a neighbouring grain partially illuminated by the laser beam). Figure 2: Spectra of photogenerated longitudinal and TA modes for different crystallographic orientations. Transient optical reflectivity signals obtained for different grains of the polycrystalline BFO sample with pump (probe) wavelength of ( a ) 415 nm (590 nm) and ( c , e ) 400 nm (800 nm). The Brillouin oscillations (BO) are clearly visible. The Brillouin signal exhibits deep dependence on the grain while the electronic excitation (EE) is independent. ( b , d , f ) Plots of the corresponding fast fourier transforms of signals shown in ( a , c , e ). The grain 1–4 are inclined grains versus z axis of the unit cell of BFO and show clear shear TA modes. ( g , h ) Sketches of the mean macroscopic polarization P direction relative to the grain surface normal n . The surface orientation of grain 2 is indicated on the mosaic (inset of g ) as an example. Grain 5 has its z axis (called optical axis) parallel to the grain surface and TA modes are nearly absent, while LA modes are visible with a splitting due to optical anisotropy of BFO (see Methods). The family of planes, to which belongs the surface of grain 5, is indicated with the black line on the mosaic (inset of h ) (remark: the small signal at ~30 GHz for grain 3 is an artefact probably arising from a neighbouring grain partially illuminated by the laser beam). Full size image Such giant amplitude of shear mode compared with that of LA one, has never been observed up to now in any materials (see Table 1 ) [22] , [23] , [26] . Indeed, in most of metals and semiconductors, the magnitudes of TA phonons are usually much weaker than that of the simultaneously generated LA phonons, which in some applications is a major drawback. Different approaches have been considered to enhance the TA response by either playing with inverse piezoelectric effect [35] or by introducing an anisotropy through special materials design, including asymmetrically cut surfaces [22] , [23] , [26] , or asymmetric multiple quantum wells embedded in p – n semiconductor junction [25] . Despite these various strategies, the shear TA phonon compared with the longitudinal LA one does not exceed 1, while here using bulk BFO ferroelectric oxide a ratio up to 6 can be achieved depending on the grain orientation ( Table 1 ). Ferroelectric oxides offer an easy and efficient way to obtain high shear responses as well as various ratio of intensity signal between TA and LA modes. Photogeneration and photodetection processes characteristics It is now of interest to analyse the behaviour of both photo-induced LA and TA modes depending on the light parameters used during the excitation and detection processes. 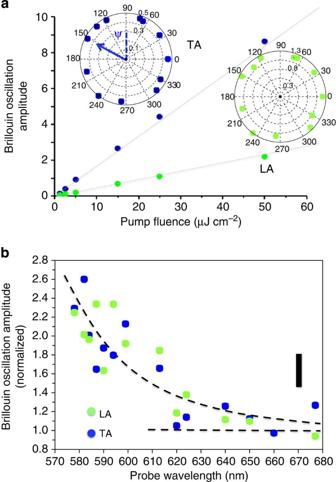Figure 3: Characteristics of ultrafast optical generation and detection processes. (a) Example of pump fluence dependence of the LA and TA mode for grain 3 (pump polarization dependence is given in inset). (b) Probe wavelength dependence of the amplitude of both TA and LA modes. For a clarity of comparisons, the LA and TA signal amplitudes are normalized by their minimum detected values. The typical error bar on the acoustic mode amplitude is given by the solid vertical segment. Figure 3a shows typical evolution of the Brillouin oscillation amplitude as a function of the pump fluence. This Brillouin amplitude exhibits a linear response for LA modes, in agreement with previous observations [35] , as well as for TA modes. Figure 3: Characteristics of ultrafast optical generation and detection processes. ( a ) Example of pump fluence dependence of the LA and TA mode for grain 3 (pump polarization dependence is given in inset). ( b ) Probe wavelength dependence of the amplitude of both TA and LA modes. For a clarity of comparisons, the LA and TA signal amplitudes are normalized by their minimum detected values. The typical error bar on the acoustic mode amplitude is given by the solid vertical segment. Full size image This linear evolution contrasts strongly with the non-linear behaviour found in piezoelectric semiconductors [22] , [23] , [24] or in PbTiO 3 ferroelectric material [42] , which was explained by a non-linear inverse piezoelectric response. Inset in Fig. 3a shows the amplitude response for different polarizations of the pump beam electric field. For both TA and LA modes, no detectable change is observed with light polarization precluding electrostriction effect as an important mechanism for acoustic wave photogeneration [19] . It is worth noting that a dependence of the lattice volume on the polarization of the incident pump light has been found in BFO single crystal in a photostriction measurement. However, this latter study, in contrast to our experiments, has been performed under a nearly static optical excitation regime [34] . Figure 3b displays the probe wavelength dependence of phonon amplitude signal during the detection process between 580 and 680 nm. The amplitude of both LA and TA modes increases monotonously by decreasing the wavelength value towards the gap value (~460 nm). This is generally expected and well known for semiconductors [21] as the efficiency of the detection increases when the probe wavelength approaches an interband optical transition. Among possible mechanisms driving the ultrafast coherent phonons emission, our data exclude any major electrostriction contribution. Moreover, thermoelastic process has been ruled out by recent time-resolved X-ray diffraction measurements [35] . Therefore, it remains to explore the deformation potential mechanism as well as the inverse piezoelectric effect [24] . As the photo-excited carriers have a pretty long lifetime of the order of 1 ns [40] , we can assume that the deformation potential parameter is controlled by the out-of-equilibrium carriers accumulated at the bottom and top of the conduction and valence band, respectively. Consequently, the photo-induced longitudinal deformation potential parameter becomes [1] , [21] as estimated from the pressure ( P r ) dependence of the direct band gap E g [43] . It is worth mentioning that this extracted value corresponds to an averaged value of the deformation potential contribution in the three crystallographic directions with . This modest value of ā is twice smaller than that of piezoelectric GaAs semiconductor with and more remarkably it is of opposite sign [21] . The negative value indicates that the photo-induced stress driven by longitudinal deformation potential is a compressional stress, and thus due to the electronic pressure the photo-excited lattice should contract. This is in complete contrast with recent observations evidencing rather a lattice expansion [35] . Given a photo-excited carrier concentration of N ~5 × 10 18 −5 × 10 19 cm −3 and a bulk modulus B ~80 GPa [44] , the longitudinal deformation potential stress [1] , [21] is estimated to be . In the pseudo-cubic approximation we have , which leads to , as known for semiconductors [22] , [23] , and thus the shear electronic stress is negligible compared with the longitudinal one. Let us now estimate what would be the stress generated by the inverse piezoelectric effect. If we consider the photo-excited carriers are rapidly accelerated by the internal electric field arising from the spontaneous polarization, then these photo-induced charges will partially screen the electric field E . Therefore, one can consider a simple capacitor such as E = eN S / εε 0 , where N S is the surface density of photo-excited carriers, e the elementary electrical charge, ε 0 the dielecric constant of vacuum and the bulk BFO dielectric constant ε ~45 (ref. 45 ). For a fluence range of 10–100 μJ cm −2 , the surface density can be estimated to N S =2 × 10 13 −2 × 10 14 cm −2 , which is smaller but comparable to the surface density N S ~ P / e ~6 × 10 14 cm −2 due to P the spontaneous polarization. The photo-induced electric field becomes then E ~10–100 kV cm −1 , which leads to an inverse piezoelectric stress of σ PE = ēE ~0.3 × 10 7 −3 × 10 7 Pa using an average piezoelectric coefficient value of ē ~3 C m −2 knowing that e 33 ~2–4 C m −2 (ref. 46 ) and e 31 ~ −2.8 C m −2 (ref. 47 ). This indicates that the shear and longitudinal inverse piezoelectric stress should have the same order of magnitude , which deeply contrasts with the situation for deformation potential stress, that is, . Therefore, the observed large shear TA signal is very likely to be more dominated by a photo-induced inverse piezoelectric effect rather than driven by a shear electronic stress mechanism. As already mentioned, the largest shear mode amplitude is observed for grains where only one TA mode is observed while the LA mode magnitude is pretty weak. This peculiar situation is found for several grains and whatever the probe wavelength is (see grains 2 and 3 in Fig. 2 ). The existence of only one TA mode indicates, from symmetry principles, that the coherent acoustic phonons propagate along a direction lying into the Oyz plane of symmetry (see axis convention in Fig. 1a ). Thus Oyz plane must be perpendicular to the illuminated surface. Taking grain 2 as the reference grain for this peculiar situation and using the Brillouin frequencies experimentally obtained in Fig. 2 , we estimate the LA and TA sound velocities to be V LA ≈5,000±100 m s −1 and V TA ≈2,000±100 m s −1 . A zoom on the fast Fourier transform (FFT) obtained for grain 2 is given in Supplementary Fig. 3 . Solving the dynamic matrix (see Supplementary Note 1 ), it is then possible to estimate the values of the sound velocities for variable angle θ as shown in Supplementary Figs 4 and 5 . Taking into account not only the absolute values of the sound velocities but also the ratio of them ( Supplementary Fig. 6 ) to refine the angle value of θ , it is found that the coherent acoustic phonons emitted from grain 2 propagate along a direction that is inclined regarding to the z axis with a possible angle of θ ~−70° or ~110°. Although this angle is an approximate, it indicates that the polarization vector P is inclined regarding to the illuminated surface (as sketched in Fig. 2g ). Moreover, this result is consistent with the fact that no shear component generated by the inverse piezoelectric effect is expected as soon as the normal vector n (see Fig. 1a ) of the illuminated surface is along y axis ( θ =90°), that is, P ⊥ n , or along the z axis ( θ =0°), that is, P // n according to equation (1) obtained by tensorial calculations within 3 m point group (see Supplementary Note 2 ). Based on equation (1), it can be seen that the intensity of the shear stress generated by the inverse piezoelectric effect for this particular case of propagation inside the Oyz plane can be modulated by varying θ angle with a maximum reached for θ =45°. It is worth mentioning that e 31 and e 33 have opposite sign; hence, both contributions add for the shear stress (equation (1)). Equivalent expression of the photo-induced stress involving the longitudinal inverse piezoelectric stress and the deformation potential mechanism can be also established (see Supplementary Note 2 ). In that case, because of opposite sign of e 31 and e 33 , the longitudinal piezoelectric stress is the result of two competing terms while that of shear component (equation (1)) is the result of additive terms. This probably have an important role in the experimental observations. The generation mechanism can be also analysed for a completely different grain orientation where the optical axis ( z axis) is now parallel to the grain surface (case of grain 5, see Fig. 2e,f ). A similar calculation detailed in Supplementary Note 2 indicates that the shear component is not excited ( σ T =0) through the inverse piezoelectric effect in that particular case in good agreement with the experimental observation. These results open a path for tailoring the acoustic spectrum by the sample crystallographic orientation and should open new perspectives similar to the development of versatile GHz shear emitters. By light focusing on a grain of appropriate orientation, a desired ratio TA/LA signal can be selected. As a summary, we have shown that very efficient opto-acoustic coherent shear phonons can be observed in BFO using appropriate crystallographic orientation. Our experimental observations and their theoretical analysis indicate that this spectacular effect never observed in any materials up to now is likely to be mainly driven by inverse piezoelectric effect. This remarkable ability to light-induce shear strain makes BFO a very interesting optically triggered GHz shear strain generator and opens the path towards more efficient tools for diagnostics, for example, of biological systems, where shear responses are desired, and for tuning other properties being strain sensitive, for example, magnetic or electronic functions. Moreover, these results highlight the relevance of ferroelectrics and/or multiferroics for efficient acoustic wave generation and should encourage materials science community, including acoustic, optoelectronic or oxytronic to further explore such ferroic materials. In particular, we would like to stress on the potential interest of the new ferroelectrics family (BiT, KNN and KNO) that exhibit small and controllable band gap [48] , [49] . Beyond their interest for photovoltaics, these small band gap ferroelectrics should provide easy way to trigger lattice coherent motion with modest pump photon energy. As an additional perspective, as THz intrinsic dynamics of the internal electric fields has been already proved in ferroelectrics by electromagnetic measurements, the photo-induced generation of THz acoustic waves in ferroelectrics should be accessible in the future [31] , [32] , [50] , [51] . Sample preparation and characterizations BFO powders were synthesized by conventional solid-state reaction by mixing in stoichiometric proportions high-purity bismuth oxide Bi 2 O 3 and iron oxide Fe 2 O 3 as starting compounds. Two consecutive calcinations in air at T =800 °C for 2 h are needed to obtain the pure perovskite BFO, free from any impurity phase. The as-grown powders were then pressed to get a pellet, which was heated in air at T =800 °C for 2 h to finally obtain a BFO ceramic. The surface of the polycrystalline sample has been prepared by fine mechanical polishing method followed by a thermal treatment in air at 750 °C to relax any residual stresses. We checked that this treatment does not affect the photoacoustic response. The grains distribution at the surface of the specimen has been determined by using EBSD technique. The EBSD image reveals that the grains have a random distribution of their crystallographic orientations, as depicted in Supplementary Fig. 1 through grains of different colours. The EBSD images were carried out with a Leo Gemini 1530 Carl Zeiss field emission high-resolution scanning electron microscope. EBSD experiments were performed at a 70° detector position to sample surface and with a gun lens acceleration voltage of 20 kV. These measurements were carried out and analysed using the EDAX Orientation Imaging Microscopy software v7 (ref. 52 ). EBSD patterns were collected following a scanning routine with different step size for large and reduced areas of the sample surface. To deduce the local crystal orientation, each pattern was indexed according to the bulk R3c BFO unit cell (hexagonal lattice a =0.5588, nm, c =1.3867, nm, point group [C3v][3m]). Resulting EBSD mappings are depicted in Fig. 1b and with a larger spatial scale in Supplementary Fig. 1 , where the inverse pole figures (in colour scale, see the mosaic inset for crystal orientation in rhombohedral notation) is overlapped to the images topography (in grey scale, dark grey indicating the largest error found when indexing using the BFO reference unit cell). From these maps we can confirm that every grain presents a given crystal orientation within the confidence allowed by the EBSD pattern indexing and that no preferential orientation is seen in this ceramic sample. Raman spectroscopy studies have also been carried out on the BFO ceramic to study the structure and to illustrate that each single grain behaves like a single crystal and thus has its own crystallographic orientation ( Supplementary Fig. 2 ). The Raman experiments were conducted using a Labram Horiba Jobin Yvon spectrometer using a 632.8-nm laser and a × 50 objective lens having a numerical aperture 0.5. Typical spectra on single grains are depicted in Supplementary Fig. 2 , using analyser/polarizer parallel and perpendicular configurations. These spectra are characteristics of bulk rhombohedral BFO. The change from parallel to perpendicular polarization configurations shows a strong variation in the intensity of some modes (see Supplementary Fig. 2 ), which is a clear feature attesting that each grain behaves similar to a single crystal. Ultrafast optical measurements Each grain undergoes an above band-gap photoexcitation by a near-ultraviolet pump radiation 400 (or 415 nm) obtained by second harmonic generation of the 800 nm (or 830 nm) femtosecond laser harmonic in a BBO crystal. At these optical wavelength, the pump beam penetration depth is around 40–50 nm [28] , taking a BFO direct band gap value of around 2.6–2.8 eV [28] . The pump photogenerated acoustic phonons then create a strain field that propagates inside the grain and modulates the refractive index. In turn, the refractive index modulation disturbs the optical reflectivity of the probe beam through acousto-optic effect. Thanks to a control of the time arrival of the probe beam relative to the excitation by the pump beam, it is possible to monitor in time the transient optical reflectivity of each BFO grain and then detect the propagation of the photogenerated acoustic phonons. This detection of the emitted coherent acoustic phonons is made with a probe radiation ranging from 560 to 800 nm given, either by the femtosecond laser (800 nm) or, for the optical range 560–700 nm, by an optical parametric oscillator synchronously pumped by the femtosecond Ti:Sa laser pump. In all the experiments, the probe polarization was circular and the incident probe beam was normal to the illuminated surface. As the pump beam diameter is significantly larger than the acoustic wave length at Brillouin frequency, the diffraction length significantly exceeds the depth of the optically probed region and the acoustic waves can be considered as plane waves. Due to momentum conservation during the interaction between the probe light and acoustic phonons, only the acoustic phonon component with the Brillouin frequency f B is efficiently detected [1] . In normal incidence, the Brillouin frequency is f B =2 V s n / λ , where λ , n and V s are the probe wavelength in vacuum, the refractive index of BFO at the wavelength λ and the sound velocity of the detected longitudinal or TA phonons. For the experimental signal, this corresponds to a sinusoidal modulation of the optical reflectivity Δ R in the time domain (see Fig. 2 ). Depending on the grain orientation, some optical birefringence has to be taken into account and leads to a splitting of the Brillouin mode. The effect of the Brillouin frequency splitting is the largest when the optical axis is parallel to the surface. For the grain 5 ( Fig. 2e,f ) belonging to this limit case, the ratio between the Brillouin frequencies detected with either extraordinary ( n e ) or ordinary ( n o ) optical refractive indexes is f e / f o = n e / n o . Our experimentally determined ratio of split frequencies is very close to the known [41] ratio of the refractive indexes where we effectively obtain f e / f o ≈ n e / n o ≈0.92 with f o ≈37.3 GHz, f e ≈34.5 GHz, n o ≈2.8 and n e ≈2.6 (ref. 41 ). How to cite this article: Lejman, M. et al. Giant ultrafast photo-induced shear strain in ferroelectric BiFeO 3 . Nat. Commun. 5:4301 doi: 10.1038/ncomms5301 (2014).